The role of protein clearance mechanisms in organismal ageing and age-related diseases The integrity of the proteome, or proteostasis, is challenged during the ageing process. Damaged proteins accumulate as a consequence of ageing and may ensue from the accumulation of reactive oxygen species and a progressive decline in the ability to maintain a functional proteome [1] . This demise in proteostasis is considered one of the hallmarks of ageing [1] and contributes to multiple age-related diseases such as Alzheimer’s (AD) [2] , Parkinson’s (PD) [3] or Huntington’s disease (HD) [4] . Proteostasis is maintained by a network of cellular mechanisms that monitors folding, concentration, cellular localization and interactions of proteins from their synthesis through their degradation [5] . Chaperones assure the proper folding of proteins throughout their life cycle and under stress conditions but their activity declines with age (reviewed in refs 6 , 7 , 8 , 9 , 10 ). When the activity of chaperones is insufficient to maintain proteome stability, misfolded proteins may accumulate and impair cell function and tissue homeostasis. Damaged, misfolded, aggregated or unnecessary proteins are scavenged by the proteasome or through autophagy-lysosome [11] . The ubiquitin–proteasome system (UPS) is a complex mechanism where proteins are first targeted for degradation by the ubiquitination machinery and then recognized, unfolded and proteolyzed by the proteasome [12] . In autophagy-mediated proteolysis, proteins are degraded by the lysosome. Although lysosomal proteolysis was initially considered to be a non-selective system, it has been shown that chaperones and other cargo-recognition molecules such as ubiquitins determine the degradation of specific proteins by the lysosome [11] , [13] , [14] . Therefore, the proteasome and autophagy might be interrelated by using ubiquitin as a common marker for proteolytic degradation [11] , [13] , [14] . Both proteasome functionality and autophagic-lysosomal potential decline during the ageing process and this failure contributes to the development of age-related diseases [11] , [15] . Here we discuss the mechanistic links between protein clearance mechanisms, ageing and neurodegenerative diseases. We further describe how longevity-promoting pathways modulate the proteostasis network, providing increased stability of the proteome and protecting from the symptoms associated with neurodegenerative diseases. In this section, we review the molecular mechanisms underlying the two main protein clearance mechanisms of the proteostasis network. The proteasome The UPS is the primary selective proteolytic system in eukaryotic cells [15] , a precise mechanism that maintains the proper concentration of many regulatory proteins involved in multiple biological processes ( Fig. 1 ). In addition, the UPS is a key component of the proteostasis network to terminate damaged proteins [11] . After sequential conjugation of ubiquitins, proteins are recognized by the proteasome, which is responsible for their degradation. The proteasome is formed by the assembly of several subunits [12] ( Fig. 1 ). The core particle (20S) of the proteasome exhibits a barrel-like structure in which the 28 subunits are assembled into four seven-membered rings [12] . The two outer rings are composed by seven α-subunits (named α1 to α7), while the two inner rings are composed by seven β-subunits (β1-β7) [12] . β-rings contain the proteolytic active sites: β1, β2 and β5 present caspase-like, trypsin-like and chymotrypsin-like activities, respectively [12] . A specialized form of the 20S proteasome, known as the immunoproteasome because of its prevalence in antigen-presenting cells, is generated by replacement of the catalytic subunits by β1i, β2i and β5i (ref. 16 ). β5t, a homologue of β5, is exclusively found in the thymus and its incorporation to the proteasome reduces chymotrypsin-like activity of the proteolytic machine [17] . α-rings control the entrance of the substrate into the catalytic cavity. Although 20S particles can exist in a free form, its default status is closed and requires the binding of proteasome activators to degrade polyubiquitylated proteins. Therefore, 20S particles are considered to be inactive, unable to degrade polyubiquitylated proteins [16] . However, free 20S particles have a detectable activity independent of ATP/ubiquitination and could play a significant role in the degradation of oxidized proteins [15] , [18] . Oxidative modification is a signal for proteolysis by 20S, a process that could gain relevance with age. 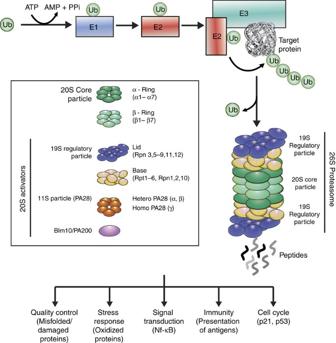Figure 1: The ubiquitin–proteasome system (UPS). Degradation by the UPS is initiated by the conjugation of ubiquitin, a highly conserved 76 amino-acid residue polypeptide, to the substrate protein12. The attachment of a ubiquitin molecule is achieved through an enzymatic sequential mechanism involving three distinct classes of enzymes12. First, the ubiquitin-activating enzyme (E1) activates the carboxyl-terminal glycine residue of a ubiquitin in an ATP-dependent manner. Activated ubiquitin is next transferred to a cysteine site of a ubiquitin-conjugating enzyme (E2). In the third step, a ubiquitin ligase (E3) links ubiquitin from the E2 enzyme to a lysine residue of the target protein. While apparently there are only two E1’s, there are several E2 enzymes and many E3 ubiquitin ligases, each of which recognizes one or several of specific protein motifs12. Therefore, E3 ubiquitin ligases are responsible for the selectivity of the process targeting specific proteins to degradation. The same cascade links additional molecules to the primary ubiquitin via internal ubiquitin lysines, forming a ubiquitin chain. Ubiquitin has seven lysine residues, all of which can form polymer chains. A chain of at least four lysine 48-linked ubiquitins is the primary signal for degradation, while other linear ubiquitin chains participate in different processes such as signal transduction39. After ubiquitination, the polyubiquitylated protein is recognized and degraded by the proteasome. Active proteasomes are formed by the interaction of proteasomal regulatory particles with a core particle (20S), which contains the proteolytic active sites. Free intracellular 20S are normally found in an inactive/closed state and require the binding of 20S activators to degrade proteins. The major assembly of the 20S proteasome is with the 19S regulatory protein, which recognizes the polyubiquitylated substrate, removes the ubiquitin moieties and unfolds the substrate to translocate it into the 20S proteolytic chamber. The 20S can also be activated by the PA28 complex or the Blm10/PA200 protein. Finally, the substrate is cleaved into short peptides. The proteasome is involved in a variety of cellular functions, such as quality control of the proteome, stress response or cell cycle regulation. Figure 1: The ubiquitin–proteasome system (UPS). Degradation by the UPS is initiated by the conjugation of ubiquitin, a highly conserved 76 amino-acid residue polypeptide, to the substrate protein [12] . The attachment of a ubiquitin molecule is achieved through an enzymatic sequential mechanism involving three distinct classes of enzymes [12] . First, the ubiquitin-activating enzyme (E1) activates the carboxyl-terminal glycine residue of a ubiquitin in an ATP-dependent manner. Activated ubiquitin is next transferred to a cysteine site of a ubiquitin-conjugating enzyme (E2). In the third step, a ubiquitin ligase (E3) links ubiquitin from the E2 enzyme to a lysine residue of the target protein. While apparently there are only two E1’s, there are several E2 enzymes and many E3 ubiquitin ligases, each of which recognizes one or several of specific protein motifs [12] . Therefore, E3 ubiquitin ligases are responsible for the selectivity of the process targeting specific proteins to degradation. The same cascade links additional molecules to the primary ubiquitin via internal ubiquitin lysines, forming a ubiquitin chain. Ubiquitin has seven lysine residues, all of which can form polymer chains. A chain of at least four lysine 48-linked ubiquitins is the primary signal for degradation, while other linear ubiquitin chains participate in different processes such as signal transduction [39] . After ubiquitination, the polyubiquitylated protein is recognized and degraded by the proteasome. Active proteasomes are formed by the interaction of proteasomal regulatory particles with a core particle (20S), which contains the proteolytic active sites. Free intracellular 20S are normally found in an inactive/closed state and require the binding of 20S activators to degrade proteins. The major assembly of the 20S proteasome is with the 19S regulatory protein, which recognizes the polyubiquitylated substrate, removes the ubiquitin moieties and unfolds the substrate to translocate it into the 20S proteolytic chamber. The 20S can also be activated by the PA28 complex or the Blm10/PA200 protein. Finally, the substrate is cleaved into short peptides. The proteasome is involved in a variety of cellular functions, such as quality control of the proteome, stress response or cell cycle regulation. Full size image Active proteasome exists in several forms, but its major assembly is formed through the assembly of the 20S and the 19S (26S, single capped or 30S, double capped) [12] . The 19S imparts regulation on the activity of the holo complex by recognizing, unfolding and translocating polyubiquitylated proteins to the 20S for degradation in an ATP-dependent process [12] , [19] . The 19S is composed of two subcomplexes: a base adjacent to the 20S and a lid that sits on top of the base [12] . The base contains six AAA-ATPases (Rpt1–6) and three non-ATPases subunits (Rpn1–2 and Rpn10). The lid, formed by eight subunits (Rpn3, Rpn5–9 and Rpn11–12), is critical for substrate recognition and deubiquitination [12] . In addition to regulation by 19S, the core particle can be activated by other regulatory particles such as Blm10/PA200 or PA28 (also known as 11S) [16] . These proteasome activators bind to the core particle opening the channel and promoting ATP- and ubiquitin-independent proteolytic degradation [16] . Compared with the 19S, their substrates are less clear although their biological functions are emerging. Blm10/PA200, a monomeric protein of 250 kDa, forms hybrid complexes in which it binds to one end of the 20S proteasome and the 19S to the opposite end [15] . PA28 is formed by hetero-heptameric rings of 28-kDa proteins (PA28α and PA28β) or homo-heptameric rings of PA28γ [16] . PA28αβ is inducible by interferon-γ and modulates the presentation and generation of specific viral antigens [15] . PA28γ is involved in cell cycle regulation promoting the degradation of small proteins such as p21 (ref. 15 ). It has been proposed that PA28 is involved in the degradation of oxidized proteins [18] . Oxidative stress causes a disassembly of the 26S/30S proteasome towards 20S and induces the PA28 and the immunoproteasome, forms supporting degradation of oxidized proteins. Taken together, proteasome activity is tightly modulated by a vast spectrum of proteasome regulators and conditions. Autophagy Autophagy is an intracellular catabolic process in which cytosol fractions, organelles and macromolecules are degraded through the lysosome. One of the main roles for autophagy is to act as a bulk intracellular degradation system that, on metabolic stress, such as nutrient deprivation, DNA damage, hypoxia or oxidative and endoplasmic reticulum (ER) stress, degrades many different substrates to support energy balance [20] , [21] . Although autophagy was initially described as a stress-induced mechanism, it exhibits basal activity. In addition, autophagy has a key role as a quality-control mechanism of proteins and organelles to maintain cellular homeostasis. Autophagy is emerging as a selective mechanism to degrade misfolded and aggregated proteins [13] . This function includes the degradation of aggregates of neurodegenerative-associated proteins such as tau, α-synuclein and polyglutamine-expanded proteins [22] . Specific receptors and adaptors, such as p62 (also known as sequestosome 1), recognize ubiquitinated proteins and target these substrates to the autophagy machinery [13] . Moreover, due to the capacity to engulf whole cellular regions, autophagy is critical in every process that requires extensive cellular remodelling, such as embryogenesis, cellular differentiation or cellular death [23] . Autophagy has been also implicated in both acquired and innate immunity through antigen presentation and degradation of peptides from external pathogens [24] . Lysosomes are the essential catalytic component of the autophagic degradation system. Lysosomes are single-membrane vesicles that contain a large variety of cellular hydrolases such as proteases, lipases, nucleotidases and glycosidases. These hydrolases reach their higher enzymatic activity at the acidic pH of the lysosomal lumen. Of particular interest of this review is proteolysis, which results from the combined action of endo- and exoproteases. This proteolytic activity leads to the conversion of proteins into small di- and tripeptides and free aminoacids that are released into the cytosol through permeases at the lysosomal membrane and either used to obtain energy or recycled to synthesize the novo proteins [25] . Depending on the type of cargo and delivery to lysosomes, autophagy is classified in different modalities. In mammalian cells, the best characterized types of autophagy are macroautophagy ( Fig. 2 ), microautophagy and chaperone-mediated autophagy (CMA) [14] , [23] , [26] , [27] . Macroautophagy (herein after called autophagy) is a self-catabolic process in which cytoplasm portions are engulfed into double membrane vesicles, which are named autophagosomes. About 35 genes, generically known as autophagy-related genes (ATG) ( Table 1 ), participate in autophagy [28] . Atg proteins organize into complexes that regulate each of the steps of autophagy. After the autophagosome is formed with the sequestered cargo inside, it is transported to the lysosome, where its outer membrane fuses with the lysosome membrane and both the sequestered material and the inner membrane of the autophagosome are degraded. The fusion is dependent on SNARE proteins VAMP8 and Vti1B [29] . In microautophagy, a pathway characterized to a much lesser extent, small components of the cytoplasm are engulfed directly by the lysosome membrane [14] . In CMA, particular cytoplasmic proteins are recognized by chaperones through a consensus sequence and transferred to the lysosome for their degradation via the lysosomal membrane-protein type 2A (LAMP-2A) receptor [26] . Autophagy and microautophagy can degrade both organelles and proteins, whereas CMA only participates in the degradation of proteins [26] . 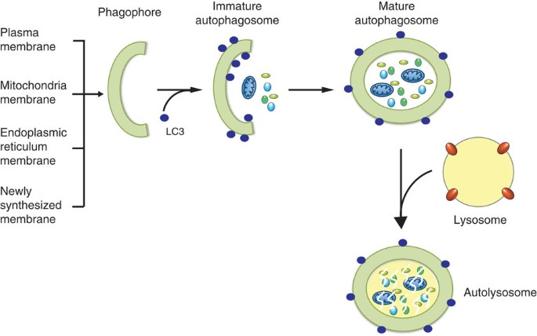Figure 2: Autophagy. Autophagy, or macroautophagy, starts with the formation of the phagophore, a double membrane that can be either newly synthesized or can be originated from the ER, mitochondria or plasma membrane. The Atg1 complex is key for the formation of the phagophore. The mammalian Atg1 homologues are the kinases ULK1 and ULK2. The ULK complex is formed, among others, by ULK1/2, Atg13 and FIP200. To promote the expansion of the phagophore, mammalian PI3K Vps34 complex—Vps15, Vps34, ATG14, Beclin-1, UVRAG, Rubicon—produces phosphatydilinositol-3-phosphate, which is crucial for the formation of the autophagosome. In the second part of the autophagic process, the cytoplasmic fraction is engulfed into the phagophore. The membrane then elongates until its edges fuse and give rise to the autophagosomes. Maturation of the phagophore comes with the conjugation of LC3 to phosphatidylethanolamine, a process known as LC3 lipidation. LC3 lipidation can occur either via assembly through the Atg12-Atg5-Atg16L complex or via processing of the newly synthesized LC3 through Atg4 to the cytosolic LC3 form (LC3I), and subsequently to the membrane binding form (LC3II). These reactions are catalyzed through Atg7 and Atg3 in a ubiquitin-like reaction. LC3II-positive autophagosomes are trafficked to the lysosomes through the microtubule network in a dynein-dependent manner. Figure 2: Autophagy. Autophagy, or macroautophagy, starts with the formation of the phagophore, a double membrane that can be either newly synthesized or can be originated from the ER, mitochondria or plasma membrane. The Atg1 complex is key for the formation of the phagophore. The mammalian Atg1 homologues are the kinases ULK1 and ULK2. The ULK complex is formed, among others, by ULK1/2, Atg13 and FIP200. To promote the expansion of the phagophore, mammalian PI3K Vps34 complex—Vps15, Vps34, ATG14, Beclin-1, UVRAG, Rubicon—produces phosphatydilinositol-3-phosphate, which is crucial for the formation of the autophagosome. In the second part of the autophagic process, the cytoplasmic fraction is engulfed into the phagophore. The membrane then elongates until its edges fuse and give rise to the autophagosomes. Maturation of the phagophore comes with the conjugation of LC3 to phosphatidylethanolamine, a process known as LC3 lipidation. LC3 lipidation can occur either via assembly through the Atg12-Atg5-Atg16L complex or via processing of the newly synthesized LC3 through Atg4 to the cytosolic LC3 form (LC3I), and subsequently to the membrane binding form (LC3II). These reactions are catalyzed through Atg7 and Atg3 in a ubiquitin-like reaction. LC3II-positive autophagosomes are trafficked to the lysosomes through the microtubule network in a dynein-dependent manner. Full size image Table 1 Summary of autophagy-related proteins. Full size table Autophagy is modulated by many signalling pathways such as adenosine monophosphate-activated protein kinase (AMPK), Sirtuin 1 (SIRT1) and mTOR, a serine/threonine kinase which exists in two complexes named mTORC1 and mTORC2. mTORC1, the mammalian target of rapamycin, can be modulated by several regulators and modulates the assembly of the Atg complex required for the formation of the autophagosomes [30] . Under fed conditions, mTORC1 is activated on the binding of growth factors to the insulin-like growth factor receptor (IGF1R), in a phosphatidylinositol 3-kinase (PI3K)/AKT-dependent manner [21] . Activated mTORC1 phosphorylates and inactivates the Atg1 complex. Conversely, under starving conditions mTOR is inhibited and the Atg1 complex consequently triggers autophagosomal vesicle formation [21] . In contrast, mTORC2 is insensitive to rapamycin inhibition and activates autophagy. Recently, unexpected findings have indicated that IGF1R depletion inhibits mTORC2 and attenuates autophagosome formation [31] . The conserved sensor of intracellular energy AMPK activates the mammalian orthologues of Atg1, ULK1 and ULK2, when the ratio AMP/ATP rises as a consequence of the energetic demand of the cell [20] . In addition, AMPK induces autophagy via the inhibition of mTOR [21] . SIRT1, a deacetylase that regulates cellular metabolism and survival, can also activate autophagy by deacetylation of several Atg proteins [32] and transcription factors, such as FOXO1,-3 and -4 (ref. 21 ). With age, post-mitotic cells lose extensive control of the proteostasis equilibrium: widespread, aberrant changes in translation, a generalized downregulation of chaperones and a loss of function in protein degradation machineries often appear in differentiated cells across time. Proteasome dysfunction during ageing can occur at different levels such as decreased expression, alteration and/or replacement of proteasome subunits [33] , [34] , [35] , disassembly of proteasomes [36] or inactivation by interacting with protein aggregates [37] , [38] . This later mechanism could induce a catastrophic proteostasis feedback during ageing, since inhibition of proteostasis itself can induce the accumulation of protein inclusions, which in turn can obstruct and further inhibit proteasome activity [37] . A decline in proteasome function during ageing and senescence has been observed in several mammalian tissues and cells such as human skin, epidermal cells, fibroblasts and lymphocytes, bovine eye lens and rat liver, lung, heart, kidney, spinal cord, hippocampus, cerebral cortex and muscle tissues [39] . Human fibroblasts are a well-established model to define senescence mechanisms. In comparison with fibroblasts that have undergone fewer passages, senescent fibroblasts exhibit a reduction in the levels of all three proteasome activities and proteasome subunit levels [40] . Several stress responses such as the heat stress response (HSR) induce the expression of chaperones to correct defects in protein folding [7] , [8] , [9] . The HSR declines with age contributing to the accumulation of damaged proteins that may overwhelm the proteolytic machinery [7] , [8] , [9] . In addition, the HSR regulates the expression of specific chaperones, such as HSP70, that bind to unfolded proteins to stimulate their degradation by the proteasome. CHIP, an E3 ubiquitin ligase, interacts with HSP70 and promotes the proteolysis of its unfolded binding partners. CHIP deficiency in mice causes a reduction in lifespan and exacerbation of ageing phenotypes, providing a link between chaperones, proteasome and ageing [41] . Similar to proteasome activity, autophagic-lysosomal potential also declines during ageing and senescence [21] , [42] . Ageing impairs autophagy of organelles, particularly that of defective mitochondria [43] , and clearance of autophagosomes with the consequent accumulation of undigested cargos inside the lysosome [44] . The molecular mechanisms mediating this demise are not fully established, although multiple studies indicate that ATG proteins, autophagy inductors and the cellular response to hormones that trigger autophagic degradation decline with age [21] . For instance, Atg5, Atg7 and Beclin-1 are downregulated in the aged human brain [45] . Furthermore, the levels of ULK1, Beclin-1 and LC3 are reduced in age-related pathologies, such as osteoarhrtitis [46] . In the liver, age-dependent decrease in autophagy may be the consequence of an inefficient clearance of the autophagosome cargo by the lysosome [44] and reduced hormonal regulation of the pathway [47] . The rate of CMA decreases with ageing [48] due to a decrease in the LAMP-2A receptor and a consequent reduction in the binding of proteins to the lysosome and their transport into the organelle [48] , [49] . The mechanism of LAMP-2A downregulation with ageing seems to be at the post-transcriptional level, since RNA levels of LAMP-2A are unchanged in ageing [49] . The heat shock protein 90 (Hsp90) is key for the assembly of LAMP-2A receptor [50] . Thus, the decline in availability of chaperones during ageing, and particularly, in Hsp90 in the aged liver [51] could explain the impairment in the trafficking and stability of LAMP-2A. Although merely correlative, these findings indicate that the loss of proteasome and autophagy may contribute to the ageing process. However, further studies in vivo are required to strengthen this potential link such as using ubiquitinated proteasome reporters or examining the autophagic flux rather than autophagosome numbers. Several genetic and functional studies have supported a casual effect of a decrease in protein clearance mechanisms and ageing. Fibroblasts treated with proteasome inhibitors have a shortened replicative lifespan and a senescent-like phenotype [52] . Knockdown of 19S and 20S subunits during adulthood shortens lifespan in Caenohabditis elegans [53] , [54] . Strikingly, a transgenic mouse with reduced chymotrypsin-like activity by replacement of the β5 subunit with β5t exhibits a shortened lifespan, premature age-related phenotypes and aggravation of age-related metabolic disorders [55] . Similarly, PA28γ deficiency promotes premature ageing in mice [56] . In yeast, a genetic screen searching for ageing factors identified multiple short-lived mutants with autophagy defects [57] . In C. elegans , decreased expression of several autophagic genes ( atg1 , atg7 , atg12 , bec1 and atg18 ) shortens its lifespan, supporting the role of autophagy in longevity [58] , [59] . In Drosophila melanogaster , the expression of autophagy genes is decreased in neurons from old flies [60] and loss of function of Atg1, Atg8 and Drosophila sestrin (dSesn, a protein required for autophagy) reduces lifespan [21] . In mice, constitutive knockout of most ATG genes is lethal during the early postnatal period due to the incapacity of energy reserves mobilization [24] . Tissue-specific deletion of several autophagy genes precipitates ageing and ageing-associated phenotypes (reviewed in refs 21 , 24 ). For instance, the central nervous system-specific knockout of Atg5, Atg7 or Atg17/FIP200 induces the accumulation of ubiquitin-positive inclusion bodies followed by neuronal loss and premature death. Purkinje cell-specific knockout of Atg7 induces axonal dystrophy and degeneration of axon terminals with a subsequent Purkinje cell death and cerebellar ataxia. It is important to highlight these findings provided one of the first direct evidences of an autophagic ubiquitinated-mediated proteolysis mechanism since neurons with compromised autophagy accumulate ubiquitinated aggregates and degenerate even with functional intact proteasomes. Autophagy dysfunction also affects other tissues. Skeletal muscle-specific knockout of Atg7 induces muscle atrophy, age-dependent decrease in force, accumulation of abnormal mitochondria, disorganization of sarcomeres and exacerbates muscle loss during denervation and fasting. Hepatocyte-specific knockout of Atg7 triggers the accumulation of lipid droplets containing triglycerides and cholesterol, induces ER stress and causes insulin stress resistance. β cell-specific deletion of Atg7 induces degeneration of pancreatic islets, impaired glucose tolerance, decreased serum insulin level, accumulation of ubiquitinylated proteins co-localized with p62, mitochondrial swelling and ER distension. Another example is the specific knockout of Atg5 in podocytes that induces spontaneous age-dependent late onset of glomerulosclerosis with accumulation of oxidized and ubiquitinylated proteins, damaged mitochondria, ER stress and podocyte loss. Different tissues exhibit different proteasome activity [61] , [62] . These findings raise the intriguing question whether the proteasome is equally affected in different cell types during ageing. This question can be addressed by using cell-specific photoconvertible reporters to measure proteasome activity in living animals [63] . A study using this methodology in C. elegans has shown that dorsorectal neurons exhibit a more severe decline in proteasome activity during ageing than body-wall muscle cells [63] . Tissue-specific differences in autophagic potential and the impact of ageing have not been systematically explored yet. The specific biological purpose of every cell type may define cellular differences in proteostasis and how ageing impacts on their protein clearance machinery. Indeed, recent findings in embryonic stem cells (ESC) support this hypothesis. ESCs do not undergo replicative senescence—a capacity that necessarily demands avoidance of any imbalance in proteostasis that would otherwise compromise its function during replication. Accordingly, human (hESCs) and mouse ESCs (mESCs) exhibit high proteasome activity compared to their differentiated counterparts and this activity does not differ depending on the passage number [64] . Increased proteasome activity is correlated with enhanced levels of the 19S subunit PSMD11/Rpn6 (refs 64 , 65 , 66 ), which is essential for the activity of the 26S/30S proteasome and stabilizes the otherwise weak interaction between the 20S core and the 19S cap [64] , [67] . Moreover, hESCs exhibit increased levels of other proteasome subunits such as α2–α5 (ref. 65 ) and the immunoproteasome subunits β1i and β5i [68] . Increased proteasome activity is required for hESC function although the reasons are unknown. Enhanced proteasome activity in these cells could be necessary to avoid senescence and maintain an intact proteome for self-renewal. Since the passage of damaged proteins to daughter cells could compromise the ageing process of an organism, increased proteasome activity could be required to generate a cell lineage with an intact proteome. Notably, the degradation of damaged proteins is triggered on the first signs of mESC differentiation via induction of PA28αβ [69] , [70] . Furthermore, both ESCs exhibit higher autophagy activity on early differentiation [71] . In addition, induced pluripotent stem cells generated from patients with PD show more autophagic vacuoles when differentiated into dopaminergic neurons [72] suggesting an active rejuvenation step to generate a pool of ‘healthy’ cells. Taken together, these results raise an intriguing hypothesis: increased proteolytic systems maintain immortality of ESCs but they are further enhanced during the initial steps of differentiation to scavenge damaged proteins that could affect the function and senescence of the new cell lineage and, therefore, organismal ageing. Once the cells are differentiated, their proteolytic potential is diminished and further reduced by the impact of ageing. Similar to hESCs, the biological function of germ line stem cells (GSCs) suggest that these cells have increased proteostasis. GSCs generate the gametes that will produce the embryos after reproduction and are designed to maintain an unlimited proliferative capacity to fulfil their biological purpose: to be passed from one generation to the next. Human oocytes and hESCs share a common transcriptome signature such as increased expression of PSMD11 (ref. 65 ). In D. melanogaster , gonads and maturating oocytes have increased 26S proteasome activity and accumulate less damaged proteins compared with ageing somatic tissues [61] , [62] . Proteasome activity is already downregulated in middle-aged flies, when signs of ageing first appear [61] , [62] . However, maturating oocytes and gonads maintain their high proteasome activity compared with age-matched somatic tissues [61] . These results support the disposable soma theory of ageing formalized by Thomas Kirkwood [73] . In this hypothesis, resources are allocated from the soma to the germline under stress conditions and ageing to prevent and repair damage to the germline. By this mechanism, the germline would ensure the fitness of the next generation. Therefore, increased proteasome activity in maturating oocytes and gonads may contribute to ensure the generation a pristine proteome in the ensuing generation. In yeast, aggregated and damaged proteins can be retained in mother cells during division [74] . In this mechanism, protein aggregates are captured by maternal mitochondria, whereas mitochondria acquired by the daughter cells are free of aggregates [75] . This asymmetric division enables the generation of a rejuvenated, germ-like, daughter cell lineage [76] . The results in flies suggest that an evolutionarily conserved mechanism may have evolved to avoid replicative senescence by establishing an ageing (soma) and rejuvenated (germ) lineage, the later with an increased proteasome activity that reduces the accumulation of damaged proteins. Adult somatic stem cell exhaustion is considered one of the tentative hallmarks of ageing [1] . These cells persist throughout the lifespan of the organism and rejuvenate tissues. However, somatic stem cell function declines during ageing in tissues such as the brain, skin, blood, bone and skeletal muscle and this failure may contribute to age-related diseases [1] , [77] . Whether adult somatic stem cells also have an enhanced proteasome activity remains to be elucidated, but the maintenance of this activity may impact organismal ageing. Experiments with adult somatic stem cells cultured in vitro such as human mesenchymal stem cells (hMSCs) [78] , haematopoietic stem cells (HSCs), dermal stem cells and epidermal stem cells [79] suggest that autophagy activity is increased in these cells compared with their differentiated counterparts. In fetal and postnatal HSCs, a deficiency in essential autophagy genes such as Atg7 or FIP200 deregulates proliferation, suggesting that autophagy is required for stemness of HSCs [80] . FIP200 is also required for neural stem cell proliferation [81] . These results suggest that autophagy could play an important role in the maintenance of specific stem cell pools. An intriguing question is whether adult somatic stem cells maintain their higher autophagy levels during organismal ageing and if a decrease in this activity could contribute to their senescence. In old mice, inhibition of mTOR with rapamycin increases lifespan and restores self-renewal of HSCs, thus improving the function of the immune system [82] . However, the impact of autophagy on the positive regulation of haematopoiesis by rapamycin is unknown. Other studies have shown that old HSCs have higher basal levels of autophagy activity and are able to induce autophagy much like young HSCs [83] . FoxO3, a forkhead transcription factor linked to stem cell maintenance and longevity [84] , maintains the expression of proautophagy genes in adult HSCs to allow a quick autophagic response on stress [83] . That old adult HSCs maintain an autophagy potential similar to young HSCs and exhibit higher levels of autophagy for their survival confronts the prevailing, traditional view where compromised autophagy is seen as a determinant of ageing [21] . Therefore, further studies are necessary to determine the links between proteolytic systems, homeostasis of stem cell pools and ageing. Gain-of-toxic-function diseases, such as AD, HD, PD and amyotrophic lateral sclerosis (ALS), in which aggregation-mediated proteotoxicity exceeds the cellular clearance machinery, are more frequent late in life even though different toxic proteins are involved in their onset [2] , [3] , [4] , [10] , [14] , [15] . The pathophysiological significance of protein aggregates is vaguely known. The accumulation of abnormal proteins may lead to perturbed cellular functions and eventually to neuronal death, ultimately manifesting as neurodegenerative disease. Unfolded monomeric proteins can be degraded through proteasome or CMA; while once aggregated into large macromolecules, bulk degradation through autophagy seems to be the key player in their removal [22] . The inclusion bodies of AD, PD, HD and ALS contain abnormal amounts of ubiquitin, suggesting a link between neurodegeneration and dysfunction of proteasome and autophagy [11] , [13] , [85] . Changes in the proteolytic machinery may explain why ageing is a risk factor for AD, PD and HD [13] , [39] , [86] . Furthermore, loss-of-function experiments have shown that decreased proteasomal activity and autophagic potential enhance the neurodegenerative phenotype [13] , [39] . In addition, there is a crosstalk between proteasome and autophagy: protein aggregation-induced proteasome or CMA impairment can activate macroautophagy, probably as a compensation mechanism [87] . Sequestration of autophagy repressors such as mTOR in protein aggregates could partially mediate autophagy induction and contribute to the typical late onset of the disease and the survival of cells with aggregates [88] . After proteasome and/or CMA failure to degrade damaged proteins, autophagy may also end up collapsing and contributing to an enhanced accumulation of aggreggates [89] . Therefore, therapies that modulate proteolytic potential may reduce aggregation-mediated toxicity. Alzheimer’s disease AD is the most common neurodegenerative disorders marked by protein aggregation and results in progressive dementia [2] . AD is characterized by the deposition of two different protein aggregates: (1) Extracellular amyloid plaques mostly formed by aggregates of β-amyloid (Aβ), which is generated via the proteolytic cleavage of the amyloid precursor protein (APP) [2] and (2) Intracellular neurofibrillary tangles mostly composed by hyperphosphorylated tau, a microtubule-associated protein [2] . Both intracellular Aβ oligomers and aggregated tau can inhibit proteasome activity [90] , [91] , which in turn could contribute to the pathology of AD. This mechanism could explain why proteasome activity is decreased in brains from AD patients compared with age-matched controls [90] . The proteasome may play a key role in delaying the accumulation of neurotoxic tau. In vitro , tau protein can be degraded by the 20S proteasome in an ATP/ubiquitin-independent manner [92] . However, other studies showed that tau proteasomal degradation is at least partially ubiquitin-dependent in cells [39] . When tau is not bound to microtubules, it associates with the chaperone Hsp70. The E3 ubiquitin ligase CHIP interacts with Hsp70 and promotes tau ubiquitination and degradation [93] . Furthermore, the inhibition of the proteasome-associated deubiquitinating enzyme Usp14 promotes tau degradation [94] . In vitro , the proteasome activator Blm10 accelerates degradation of unstructured tau [95] . Tau clearance is blocked by FK506 binding protein 51 kDa (FKBP51), which forms a chaperone complex with Hsp90 that prevents tau degradation resulting in tau oligomerization [96] . In humans, FKBP51 levels increase with age and higher FKBP51 levels are associated with AD progression [96] . Autophagy vacuoles are abundant in AD neurons and contain substantial amounts of Aβ [97] , [98] . Increased autophagy compartments occurs at early staged of the disease, when amyloid deposits are not visible [97] . Whether the autophagic flux is enhanced at this stage is unknown, although increased lysosome proliferation and lysosomal enzymes levels were observed [99] . However, autophagy declines with the disease progression contributing to the deposition of aggregated proteins [98] . In AD, both the maturation and transport of autophagosomes are impaired, and Aβ-containing autophagosomes consequently accumulate [97] , [100] . In addition, impaired lysosomal proteolysis may also contribute to Aβ accumulation. Presenilin-1, an AD-related protein involved in the early onset of the disease, regulates autophagy by acidificating autolysosomes and activating cathepsin. Presenilin-1 hypomorphic mice present impaired clearance of autophagosomes [101] . Several studies have suggested that reduced autophagy via beclin-1 contributes to the deposition of Aβ [39] . Beclin-1 expression is reduced in AD brain with age and beclin-1 deficiency reduces autophagy rate and alters APP metabolism [102] . Beclin-1 heterozygous mice present defective autophagy and neuronal degeneration, while a decrease of beclin-1 in the APP AD model enhances Aβ deposition and neuronal degeneration [103] . Parkinson’s disease PD is a neurodegenerative movement disorder characterized by the accumulation in dopaminergic neurons of Lewy Bodies [3] , which are mainly composed of α-synuclein, ubiquitin, the E3 ligase parkin and other UPS-related proteins. Soluble α-synuclein is degraded through proteasome or CMA, while once aggregated is scavenged through autophagy [104] , [105] . Several studies have suggested that proteasome dysfunction may contribute to the pathology of PD. Rats treated with proteasome inhibitors exhibit characteristics of PD, such as tremor, which is accompanied by α-synuclein and ubiquitin-containing inclusions in dopaminergic neurons [106] . However, other laboratories could not reproduce these studies [85] . In an alternative approach, conditional proteasome subunits knockout mouse models were generated since constitutive deletion is embryonically lethal [11] . Deletion of the ATPase subunit Psmc1/Rpt2 in dopaminergic neurons lead to ubiquitin and α-synuclein positive inclusions which resulted in neuronal death, thus resembling the hallmarks of PD [107] . In addition, variations in the gene PSMC4/Rpt3 correlate with the age of PD onset in patients [108] . These results suggest a role for the 26S/30S in α-synuclein degradation although it can also be degraded by free 20S in a ubiquitin-independent process [109] . Dysfunction of autophagy has also been pointed as a central pathway in the pathogenesis of PD. Mutant α-synuclein binds to the lysosome membrane with high affinity, but cannot be transported into the lysosome. Consequently, the irreversible binding of mutant α-synuclein to the lysosome blocks the binding of other substrates, resulting in a general impairment of the CMA pathway and further α-synuclein accumulation [110] . Proteins related to familiar PD, such as DJ-1 or LRRK2, significantly alter autophagy [111] , [112] . ALS is another progressive neurodegenerative movement disorder but affects motor neurons [3] . Impairment of the proteasome in these neurons by conditional knockout of Psmc4/Rpt3 revealed loss of motor neurons, locomotor dysfunction and accumulation of aggregates of TDP-43 and FUS proteins, features typical of ALS [113] . In contrast, the motor neuron-specific KO of Atg7, results in only subtle cytosolic accumulation of p62 and ubiquitin, with no TDP-43 and FUS pathologies or motor dysfunctions [113] . Therefore, under these experimental settings, proteasomal degradation appears to govern the development of ALS. Huntington’s disease HD is an autosomal dominant disease that affects muscle coordination and leads to progressive cognitive decline and psychosis [4] . HD displays selective neurodegeneration that occurs preferentially in the brain striatum [4] . The disorder is caused by the expansion of a CAG triplet repeat region in the Huntingtin gene, which translates into a polyglutamine (PolyQ) stretch in the amino-terminal domain of the protein resulting in fibril formation and aggregation [4] . An expansion of glutamines of over 40 can trigger the development of HD. Huntingtin inclusions contain ubiquitinated proteins, chaperones and components of the proteasome [114] . Proteasome activity is reduced in brains from HD patients and mice models [115] . In contrast to the soluble form of huntingtin, the aggregated form has been found to be ubiquitinated itself, suggesting an impairment of the capacity of the proteasome to degrade aberrant huntingtin [115] . Nevertheless, whether the formation of inclusion bodies in neurons is protective or toxic is still under debate. Considering the correlation between behavioural deficits and the load of misfolded huntingtin in HD mouse models, the inclusions themselves have been proposed to be on the base of the toxicity in neurons [114] , [116] . The exact mechanisms of this toxicity, however, remain unsolved but a general impairment of the proteasomal function resulting in proteostasis collapse and cellular death has been proposed [117] . An in vitro study suggested that the proteasome is not able to cleave within PolyQ stretches and the occasional failure of these long undegradable sequences to exit the proteasome may interfere with its function [118] . Accordingly, incubation of proteasomes with mutant huntingtin exerts an inhibitory effect on the proteasome by directly impeding the entrance of other substrates [119] . However, other studies found that huntingtin aggregates do not affect proteasome activity suggesting that proteasomal dysfunction may be a consequence of a general proteostasis collapse [120] , [121] . Huntingtin aggregates can be degraded through autophagy [122] and autophagy inhibition enhances the disease [88] , [123] , [124] . Autophagy dysfunction seems to play an important role in HD but the molecular bases underlying this mechanism have not been fully elucidated. In cells from HD patients and HD mouse models, a defect in the effective cargo recognition by autophagosomes was demonstrated [125] . In addition, mutant huntingtin can sequester beclin-1, and consequently inhibit autophagy, what further enhances huntingtin accumulation [126] . Age-induced reduction in beclin-1 expression would also contribute to the major accumulation of huntingtin in old neurons [126] . Wild-type huntingtin participates in the induction of autophagy on ER stress whereas mutant huntingtin-expressing cells have a perturbed ER function and increase autophagosomes [127] . Furthermore, decreased dynein function impairs autophagic clearance of aggregate-prone proteins and enhances the toxicity of the mutation that causes HD in fly and mouse models [128] . Cancer Ageing is a primary risk factor for cancer [1] , [129] . Cancer is the consequence of an aberrant gain of cellular fitness, whereas ageing is characterized by a loss of fitness. Although ageing and cancer may seem to be opposite processes, both can share common origins: the cellular damage accumulated during ageing triggers cellular senescence, but this damage occasionally provides aberrant advantages to specific cells [1] , [129] . Several studies have suggested that proteasome activity is elevated in human cancers [39] . The high degree of cell division and high mutation rates in cancer cells lead to an accumulation of misfolded proteins, which activate stress responses and/or apoptosis. The upregulation of proteasomal activity may eliminate these aberrant proteins that otherwise would be toxic for the cell [130] . Proteasome activity could have an important role in theories that suggest a relationship between the onset of cancer and ageing of somatic stem cells [129] . During ageing, these cells accumulate DNA damage from stress such as intracellular oxidants. Typically, these damaged cells undergo cell arrest, apoptosis or senescence decreasing homeostasis of stem cell pools. However, some rare cells can escape from the default pathway, acquiring additional mutations that allow them to proliferate and increase the likelihood of cancer [129] . Thus, a better knowledge of how somatic adult stem cells regulate their proteasome activity may help to understand the origin of cancer stem cells and find specific treatments. Whether proteasome modulation would result in selective inhibition of malignant cell growth is unclear, but proteasome inhibitors have become valuable tools in the treatment of certain types of cancer [39] . The underlying mechanisms for this selectivity might be that malignant cells show greater sensitivity to the cytotoxic effects of proteasome inhibition than non-cancer cells [39] . Likewise, immortal hESCs are more sensitive to proteasome inhibition than their differentiated counterparts [64] . In contrast, increased autophagy plays an important role in oncogenic suppression since its inhibition increases the frequency of tumours in mice [21] . Autophagy regulators such as beclin-1, Atg4c and AMBRA1, act as oncosuppressors since their loss increases the frequency of tumours in rodents [131] . Removal of the oncogenic protein p62 induced by autophagy suppresses oncogenesis [132] . In addition, autophagy is upregulated during and partially required for oncogenic Ras-induced senescence and apoptosis limiting the oncogenic potential of deregulated Ras signals [133] , [134] . Enhanced proteasome activity and/or autophagy extend longevity. Here we discuss recent insights into the activation of protein clearance mechanisms induced by longevity-promoting pathways. Increased protein clearance mechanisms extend healthspan Several reports suggest that sustained proteasome activity correlates with longevity. Notably, proteasome activity is increased in long-lived humans (centenarians) [135] . In this study, the levels of proteasome subunits and proteasome activity were analysed in fibroblasts derived from healthy centenarians and compared with fibroblast from young and old control donors. Strikingly, proteasome subunits and activity levels in healthy centenarian-derived fibroblasts are more similar to the younger than the older control donor-derived fibroblasts [135] . Furthermore, increased proteasome activity was found in extremely long-lived animals such as the naked mole rat [136] and the giant clam [137] . This link between increased proteasome activity and longevity has been further supported by genetic approaches ( Fig. 3a ). In Saccharomyces cerevisae , overexpression of the proteasome chaperone UMP1/POMP induces an enhanced preservation of proteasome-mediated proteolysis and increased viability during stationary-phase, a model for post-mitotic ageing [138] . In yeast, Rpn4 acts as a transcription factor regulating the levels of proteasome subunits and promoting proteasome activity [139] . Rpn4 degradation is promoted by the E3 ubiquitin ligase Ubr2. Loss of UBR2 results in elevated levels of Rpn4 and increased replicative lifespan and resistance to proteotoxic stress in yeast [140] . Ectopic expression of 19S proteasome subunits extends lifespan in invertebrates. A genetic gain-of-function screen in D. melanogaster showed that Rpn11 overexpression suppresses the age-dependent reduction of 26S/30S proteasome activity and extends lifespan, whereas rpn6 overexpression increases longevity in worms [141] . Furthermore, increased assembly of active proteasomes induced by the overexpression of β5 or POMP confers resistance to oxidative stress and delays senescence in human fibroblasts [142] . 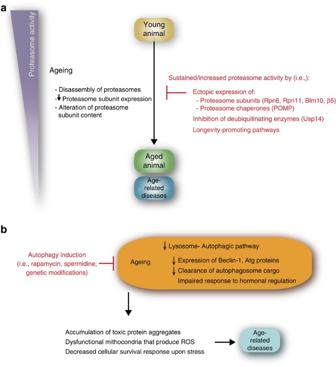Figure 3: Links between protein clearance mechanisms and ageing. (a) Proteasome activity declines with ageing as a consequence of a reduction in the expression of proteasomal subunits, alteration or replacement of several proteasomal subunits, disassembly of the proteasome or inactivation of the proteasome through direct interaction with age-induced protein aggregates. Consequently, interventions that increase and sustain proteasome activity such as the overexpression of proteasome subunits and chaperones can extend lifespan and delay the onset of age-related diseases. Several longevity-promoting pathways (that is, DR or reduced insulin/IGF-1 signaling pathway (IIS)) increase proteasome activity. Likewise, long-lived organisms (that is, the naked mole rat and the giant clam) and centenarians exhibit increased proteasome activity. (b) Autophagy declines with age as a consequence of reduced expression of autophagy-related proteins, decreased clearance of autophagosomes cargo or impaired response to hormonal regulation. Activation of autophagy, either pharmacologically or genetically, promotes longevity and delays the onset of age-related diseases. Figure 3: Links between protein clearance mechanisms and ageing. ( a ) Proteasome activity declines with ageing as a consequence of a reduction in the expression of proteasomal subunits, alteration or replacement of several proteasomal subunits, disassembly of the proteasome or inactivation of the proteasome through direct interaction with age-induced protein aggregates. Consequently, interventions that increase and sustain proteasome activity such as the overexpression of proteasome subunits and chaperones can extend lifespan and delay the onset of age-related diseases. Several longevity-promoting pathways (that is, DR or reduced insulin/IGF-1 signaling pathway (IIS)) increase proteasome activity. Likewise, long-lived organisms (that is, the naked mole rat and the giant clam) and centenarians exhibit increased proteasome activity. ( b ) Autophagy declines with age as a consequence of reduced expression of autophagy-related proteins, decreased clearance of autophagosomes cargo or impaired response to hormonal regulation. Activation of autophagy, either pharmacologically or genetically, promotes longevity and delays the onset of age-related diseases. Full size image Activation of autophagy, either pharmacologically or genetically, promotes longevity in C. elegans [143] , D. melanogaster [144] and mice [145] ( Fig. 3b ). Rapamycin treatment extends longevity in invertebrates and mammals [21] . However, due to the multiple targets of mTOR, it cannot be ruled out that other autophagy-independent pathways, such as the immune environment or regulation of protein translation, could be also involved in rapamycin-induced longevity [146] . Strikingly, enhanced expression of Atg1, Atg8 and dSesn promotes longevity in flies [21] and overexpression of Atg5 increases autophagy and extends lifespan in mice [147] . Furthermore, an increase in the levels of LAMP-2A prevents ageing-associated dysfunctions in the liver of old mice [148] . In C. elegans , enhanced autophagy via overexpression of the basic helix–loop–helix (HLH) transcription factor EB (TFEB) extends lifespan [149] . TFEB/HLH-30 induces many autophagy and lysosomal-related genes [150] . However, the longevity phenotype induced by TFEB/HLH-30 is caused by increased lysosomal lipolysis and might be independent of proteostasis [149] , [151] . Multiple studies have shown that increased clearance mechanisms ameliorate age-related diseases. Enhancement of the proteasome machinery has been proven beneficial in HD models. Increased levels of Rpn6 in C. elegans or Rpn11 in D. melanogaster reduce toxic aggregates and suppress expanded PolyQ-induced neurodegeneration in HD models [54] , [141] . Increased expression of PA28γ improves cell survival in a cellular model of HD [152] . Modulation of autophagy has beneficial effects on neurodegenerative diseases. In flies and mouse models of AD, activation of autophagy by rapamycin treatment increases clearance of tau and Aβ aggregates [153] , [154] . Likewise, activation of autophagy by rapamycin treatment increases clearance of α-synuclein aggregates in cells that express mutant α-synuclein [105] . The overexpression of beclin-1 ameliorates the accumulation of α-synuclein by enhancing lysosomal function and reducing the deficits in the autophagic pathway [155] . Pharmacological autophagy activation also ameliorates HD phenotype [88] , [123] , [124] . Reduced insulin/IGF-1 signalling Reduced insulin/IGF-1 signalling (IIS) promotes longevity and increases stability of the proteome, which delays the onset of age-related diseases [10] . Reduced IIS extends lifespan in both invertebrates and vertebrates [156] and correlates with increased longevity in humans [157] , [158] . The insulin/IGF-1 receptor activates a conserved PI3-kinase /PDK/AKT signalling cascade that phosphorylates FOXO transcription factors, thereby preventing their nuclear localization. When IIS signalling is reduced, FOXO accumulates in the nucleus and regulates downstream genes that extend lifespan and increase stress resistance [156] . In C. elegans , the CUL-1 E3 ubiquitin ligase complex is required for the extended lifespan of IIS mutant worms. This regulation is achieved, at least in part, by promoting the transcriptional activity of the worm FOXO transcription factor DAF-16 (ref. 53 ). Decreased IIS induces proteasome activity in worms through DAF-16 transcriptional repression of the proteasome-associated deubiquitinating enzyme ubh-4 (ref. 159 ). UCHL5 , the human orthologue of ubh-4, increases degradation of toxic proteins in mammalian cells [159] . Autophagy also contributes to the longevity phenotype of reduced IIS C. elegans mutants. In fact, IIS worm mutants constituted the first model in which a causative effect between autophagy and longevity was shown [160] . Since then, the requirement of autophagy for lifespan extension has been demonstrated in practically all long-lived C. elegans strains such as dietary restriction (DR), mitochondrial electron transport chain, reduced TOR and germline-lacking mutant worms [149] , [161] . In this context, the transcription factor HLH-30/TFEB, which activates autophagy, may be an universal regulator of longevity since it is required for the lifespan of long-lived mutant worms [149] . In worms with mutations in the insulin receptor daf-2 , longevity is abolished and autophagosomes accumulate when autophagy is inhibited by mutation of essential ATG genes [160] . Autophagy-dependent lifespan extension requires bec1 (a beclin-1 orthologue) but not DAF-16. Nevertheless, due to the requirement of DAF-16 for lifespan extension in daf-2 mutants, autophagy is most probably not sufficient for the longevity phenotype [162] . Delayed ageing, by IIS reduction, protects from protein aggregation toxicity [163] , [164] . Experiments using C. elegans expressing polyQ in body-wall muscle showed that toxic protein aggregation is age dependent [165] . IIS reduction delays polyQ aggregation and toxicity suggesting that this pathway modulates the proteostasis network to enable cells to deal with toxic proteins to a much later age [165] . Whether reduced IIS ameliorates polyQ aggregation by modulating, at least partially, protein clearance mechanisms has not been examined. In a C. elegans model of AD, expression of Aβ 1–42 peptide in the body-wall muscle cells produces a progressive paralysis phenotype [166] . In a DAF-16-dependent manner, reduced function of the IIS can protect from the toxicity of Aβ 1–42 by inducing the aggregation of small toxic Aβ 1–42 oligomers into larger, less toxic structures [167] . These results suggest the activation of an aggregation mechanism and have been substantiated in mice, in which a heterozygous mutation in the IGF-1 receptor is protective in a mouse model of AD [164] . Autophagic degradation of Aβ is also required for the protective effect of reduced IIS in Aβ 1–42 -expressing worms, whereas the role of proteasome activity has not been examined [168] . In mice, IIS effects could be independent of autophagy since IGF1R inhibition results in decreased autophagy [31] . Besides IIS, other growth factors regulate ageing [169] . Epidermal growth factor signalling promotes longevity in C. elegans . Upregulation of both proteasome activity and polyubiquitination, and a consequent decrease in protein aggregation are required for the lifespan extension induced by epidermal growth factor signalling [170] . Signals from the reproductive system Hypothetically, the need for repairing and preventing damage to the germline dominates resource allocation strategies, while the somatic tissues age and deteriorate [73] . In support of such theory, modulations of reproduction that eliminate germ cells in C. elegans and D. melanogaster extend lifespan [171] , a phenotype that may be caused by heightened proteome stability within the post-mitotic soma [54] , [172] . Inhibiting germline proliferation induces an increased in proteasome activity and RPN6 levels in the somatic tissues and protects from polyQ-dependent aggregation [54] , [172] . Similar to immortal hESCs, increased proteasome activity, rpn6 expression and longevity are modulated by DAF-16 in these long-lived animals [64] , [173] . Interestingly, DNA damage in C. elegans germ cells induces a systemic response that protects somatic tissues by increasing their proteasome activity [174] . Furthermore, autophagy and lipase-4-dependent lypolisis modulate the longevity phenotype of germline-lacking worms in an interconnected manner [175] . This interplay occurs through a coordinated action of mTOR and PHA-4/FOXA, a transcription factor that regulates the expression of several autophagy genes. Dietary restriction Reduced food intake without malnutrition extends lifespan in multiple species [176] . DR modulates translational rates inducing a decrease in the load of nascent polypeptides to the proteostasis machinery [177] , which may allow more efficient protein folding and degradation. In mice, DR induces the expression of the 19S proteasome subunit Psmc3/Rpt5 and the proteasome activator PA28α [34] . In C. elegans , the HECT E3 ubiquitin ligase WWP-1 is a positive regulator of lifespan in response to DR [178] . This lifespan extension induced by WWP-1 is dependent on pha-4 (ref. 178 ). In addition, the oxidative stress-responsive transcription factor skn-1 is also required for DR-induced longevity in C. elegans [179] . skn-1 promotes the expression of aip-1 /AIRAP (arsenic-inducible RNA-associated protein) under metabolic stress [180] . aip-1 /AIRAP binds to the 19S increasing proteasome activity and clearance of damaged proteins [181] . Notably, aip-1 /AIRAP ameliorates Aβ and polyQ toxicity [182] , [183] . Moreover, skn-1 and its mammalian orthologues Nrf1 and Nrf2 upregulate the expression of proteasomal genes in response to proteasome inhibition and oxidative stress [39] . Inducible Nrf2 activation in D. melanogaster promotes youthful expression of proteasome subunits in aged somatic tissues [62] . This result suggests that age-dependent Nrf2 dysfunction may contribute to the decrease in proteasome subunit expression with age. Interestingly, Nrf2-mediated proteasome activation delays senescence in human fibroblasts [184] . Autophagy is required for the anti-ageing effects of DR in all the species investigated [21] . In addition, DR is sufficient to increase autophagic potential through the activation of either AMPK or SIRT1 depending on how it is applied (that is, intermittent feeding versus chronically reduced intake), its intensity and its onset [21] . DR also induces autophagy through the inhibition of IIS [143] . Similar to germline-lacking worms, DR-induced autophagy requires pha-4 , which increases the expression of ATGs [162] , [185] . Longevity-promoting pathways increase functionality of protein clearance mechanisms, which contributes to the amelioration of age-related diseases. Although related studies have been performed mostly in invertebrates, their results could be translated into a valuable therapeutic approach for the treatment of progressive, age-related neurodegenerative diseases. However, further studies in mammals are required to strengthen the potential link between increased protein clearance mechanisms and the delayed onset of age-related disorders. How to cite this article: Vilchez, D. et al. The role of protein clearance mechanisms in organismal ageing and age-related diseases. Nat. Commun. 5:5659 doi: 10.1038/ncomms6659 (2014).